Enhanced mechanical properties of nanocrystalline boron carbide by nanoporosity and interface phases Ceramics typically have very high hardness, but low toughness and plasticity. Besides intrinsic brittleness associated with rigid covalent or ionic bonds, porosity and interface phases are the foremost characteristics that lead to their failure at low stress levels in a brittle manner. Here we show that, in contrast to the conventional wisdom that these features are adverse factors in mechanical properties of ceramics, the compression strength, plasticity and toughness of nanocrystalline boron carbide can be noticeably improved by introducing nanoporosity and weak amorphous carbon at grain boundaries. Transmission electron microscopy reveals that the unusual nanosize effect arises from the deformation-induced elimination of nanoporosity mediated by grain boundary sliding with the assistance of the soft grain boundary phases. This study has important implications in developing high-performance ceramics with ultrahigh strength and enhanced plasticity and toughness. Boron carbide (B 4 C) is an important ceramic material because of low density, high Hugoniot elastic limit, super-high hardness and good electric conductivity [1] , [2] , [3] , [4] . It has been used in a variety of important applications where hardness, weight and conductivity are critical. However, the low toughness and strength as well as poor damage tolerance have limited their widespread use as structural and functional materials [3] , [4] . As strength and plasticity of brittle materials are sensitive to the fabrication flaws that may act as stress concentrators or weak points for crack initiation and thereby catastrophic failure [5] , [6] , various attempts have been made to improve the sintering density of B 4 C ceramics with different sintering additives [7] , [8] , [9] . Although those sintering aids can increase the specific density of B 4 C, the fracture toughness, ductility and strength were only improved marginally [10] , [11] . Nanocrystalline ceramics are known to exhibit numerous outstanding properties compared with conventional polycrystals [12] . In particular, these ceramics are expected to have a combination of high strength and enhanced ductility [13] . However, avoiding grain coarsening during high temperature sintering remains challenging [14] , [15] . In this article, we report the mechanical properties of nanocrystalline boron carbide (n-B 4 C) with a homogenous distribution of nano-sized pores and amorphous carbon at grain boundaries (GBs). Unexpectedly, we found that the nanopores and weak interface phases are effective in enhancing the fracture toughness, plasticity and compression strength of the brittle ceramic simultaneously. Pristine structure characterization Nanocrystalline B 4 C powders containing slightly excessive carbon, namely 2–3 vol. % higher than that of stoichiometric, were sintered at a relatively lower temperature in order to obtain a fine-grained microstructure. The relative density of the bulk n-B 4 C is 92.8% of the theoretical value; assuming 2–3 vol. % free carbon, the porosity of the sintered sample is ~8–10%. The X-ray diffraction (XRD) pattern ( Supplementary Fig. S1 ) indicates that the sample is highly crystallized B 4 C with rhombohedral structure ( space group: R 166 ) and a detectable secondary phase cannot be seen as amorphous carbon is inaccessible by XRD. The typical scanning electron microscopy (SEM) image of the fractured surface of n-B 4 C reveals nearly equiaxed grains with sizes in the range of ~40 to 150 nm ( Fig. 1a ). 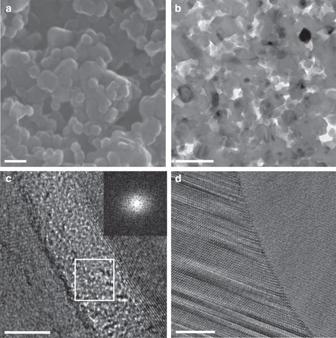Figure 1: Electron microscope characterization of as-synthesized n-B4C. (a) The SEM micrograph of as-sintered n-B4C with nanograins ranging from 40 to 150 nm. Scale bar, 100 nm. (b) TEM image of as-synthesized n-B4C. Fine pores with sizes of ~20–70 nm evenly distribute in the sample and the mean size is of ~32(±7) nm determined by an image tool analyser. Scale bar, 200 nm. (c) HRTEM image of an amorphous carbon layer between two B4C nanograins. Scale bar, 5 nm. The insert is the fast Fourier transform pattern taken from the amorphous GB phase. (d) HREM image of a clean B4C grain boundary without a detectable GB phase. Scale bar, 10 nm. Figure 1b shows the bright-field transmission electron microscopy (TEM) image of the sample, in which a high number densities of nanopores are distributed homogenously throughout the sample. The nanopores have an irregular shape with a size ranging from 20 to 70 nm ( Fig. 1b ) at GBs and GB triple junction points. The mean diameter is estimated to be ~32±7 nm, which is about half of the average grain size. High-resolution TEM (HRTEM) images show that there is a thin layer of amorphous carbon at most GBs and the internal surface of nanopores as shown in Fig. 1c and Supplementary Fig. S2 . The fast Fourier transform pattern (the inset of Fig. 1c ) further confirms the amorphous nature of the interface phase. In addition, clean GBs without detectable interface phases can also be observed by HRTEM ( Fig. 1d ). Figure 1: Electron microscope characterization of as-synthesized n-B 4 C. ( a ) The SEM micrograph of as-sintered n-B 4 C with nanograins ranging from 40 to 150 nm. Scale bar, 100 nm. ( b ) TEM image of as-synthesized n-B 4 C. Fine pores with sizes of ~20–70 nm evenly distribute in the sample and the mean size is of ~32(±7) nm determined by an image tool analyser. Scale bar, 200 nm. ( c ) HRTEM image of an amorphous carbon layer between two B 4 C nanograins. Scale bar, 5 nm. The insert is the fast Fourier transform pattern taken from the amorphous GB phase. ( d ) HREM image of a clean B 4 C grain boundary without a detectable GB phase. Scale bar, 10 nm. 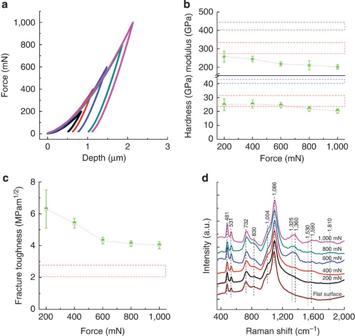Figure 2: Mechanical properties and Raman spectroscopy analysis. (a) Indentation force versus depth curves during loading and unloading with the maximum loads ranging from 200 to 1,000 mN at a constant loading rate of 7.06 mN s−1. (b) The variation of mean value of elastic modulus (E) and micro-indentation hardness (H) plots ranging from 290–200 GPa and 28–21 GPa at different loading forces (green colour). For comparison, the data taken from B4C single crystals (refs4,21,Eranging from 400–450 GPa andHfrom 40–42 GPa) and microcrystalline B4C (refs17,18,19,20,Eranging from 270–340 GPa andHfrom 25–32 GPa) are also plotted here. The data ranges marked by the dashed blue dotted lines correspond to single crystals B4C and the data ranges marked by the dashed red dotted lines correspond to microcrystalline B4C. (c) The variation of mean fracture toughness as a function of loading forces (green colour). For comparison, the data taken from microcrystalline B4C (refs18,19,20,24,25, red dotted lines) are in the range from 2 to 2.8 MPa m1/2.The measured fracture toughness of n-B4C is ~3.6–4.7 MPa m1/2,much higher than that of microcrystalline B4C. The error bars represent the standard deviation from all the ten indentations measurements. (d) Raman spectra taken from the pristine area and residual indents of n-B4C at different loads. Full size image Mechanical properties and Raman spectroscopy analysis Figure 2a shows the load-depth curves of instrumented indentation testing at a constant loading rate of 7.06 mN s −1 . All the curves are smooth without any pop-in or pop-out behaviour. The hardness ( H ) and elastic modulus ( E ), calculated according to the Oliver–Pharr method [16] , are 21–28 and 200–290 GPa, respectively. Figure 2b plots H and E as the function of the maximum applied load, P , from which the indentation size effect can be seen with lower P leading to higher H and E values. The indentation size effect is probably associated with the strain gradient underneath indenter, which may be different from the one in metals caused by geometrical necessary dislocations. The H and E values of n-B 4 C are comparable to those of microcrystalline B 4 C at similar loads [17] , [18] , [19] , [20] , but less than those of single-crystal B 4 C (ref. 21 ). The reduced hardness and elastic modulus can be attributed to the presence of nanoporosity and soft amorphous carbon at GBs in n-B 4 C. The fracture toughness of n-B 4 C was measured by nanoindentation according to the following equation [22] : Where P is the maximum indentation load, c is the crack length, E is the Young's modulus and H is the hardness; x v was determined as 0.016 by Ouchterlony [23] . The crack length c is measured from the indentation centre to the tip of the emanated cracks as shown in the inset of Supplementary Fig. S3 . The measured toughness value is ~3.6–4.7 MPa m 1/2 ( Fig. 2c ), more than 75% higher than that of microcrystalline B 4 C (refs 18 , 19 , 20 , 24 , 25 ). Figure 2d shows the typical Raman spectra collected from the pristine and residual indents at different loading forces. At low loading levels, the Raman bands extending from 350 to 1,200 cm −1 are in good agreement with the unindented spectra, and the characteristic Raman bands are located at 481, 531, 732, 830, 1,004 and 1,086 cm −1 . At the loading levels above 600 mN, intense Raman bands at 1,325 and 1,360 cm −1 , followed with short peaks at 1,530 and 1,590 cm −1 and 1,810 cm −1 , can be observed [21] , [26] , indicating partial phase transition from crystalline to amorphous boron carbide (a-B 4 C) along with the presence of amorphous carbon. Figure 2: Mechanical properties and Raman spectroscopy analysis. ( a ) Indentation force versus depth curves during loading and unloading with the maximum loads ranging from 200 to 1,000 mN at a constant loading rate of 7.06 mN s −1 . ( b ) The variation of mean value of elastic modulus ( E ) and micro-indentation hardness ( H ) plots ranging from 290–200 GPa and 28–21 GPa at different loading forces (green colour). For comparison, the data taken from B 4 C single crystals (refs 4 , 21 , E ranging from 400–450 GPa and H from 40–42 GPa) and microcrystalline B 4 C (refs 17 , 18 , 19 , 20 , E ranging from 270–340 GPa and H from 25–32 GPa) are also plotted here. The data ranges marked by the dashed blue dotted lines correspond to single crystals B 4 C and the data ranges marked by the dashed red dotted lines correspond to microcrystalline B 4 C. ( c ) The variation of mean fracture toughness as a function of loading forces (green colour). For comparison, the data taken from microcrystalline B 4 C (refs 18 , 19 , 20 , 24 , 25 , red dotted lines) are in the range from 2 to 2.8 MPa m 1/2 .The measured fracture toughness of n-B 4 C is ~3.6–4.7 MPa m 1/2 ,much higher than that of microcrystalline B 4 C. The error bars represent the standard deviation from all the ten indentations measurements. ( d ) Raman spectra taken from the pristine area and residual indents of n-B 4 C at different loads. Full size image Microstructural characterization of deformed n-B 4 C In order to determine the underlying micromechanisms accounting for the enhanced toughness of n-B 4 C, a cross-sectional TEM specimen was sliced from the residual indent using focused ion beam (FIB) milling. 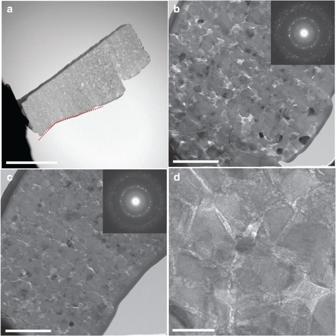Figure 3: Evidence of GB sliding within the deformed area. (a) TEM micrograph of n-B4C sliced from an indented impression made by 1,000-mN applied force. The sliced residual indent was lifted up using FIB and attached to Cu grid. The dash line (red) indicates the profile of the residual indent. Scale bar, 2 μm. (b) Bright-field TEM image of undeformed region shows the homogenous distribution of nanoporosity. The inserted is a SAED pattern taken from this region. Scale bar, 500 nm. (c) Bright-field TEM image of the deformed area (underneath the indenter) showing the elimination of nanoporosity. The inserted SAED pattern is taken from the deformed region with densely distributed rings owing to increased nanograin density. Scale bar, 500 nm. (d) Zoom-in TEM image beneath indenter showing the well-distributed amorphous phases along GBs caused by GB sliding. Scale bar, 50 nm. Figure 3a shows a TEM micrograph of the indented region at the maximum load of 1,000 mN. It can be seen that both the population and size of the nanopores have been reduced by the external loading force and the structure has been densified in comparison with the neighbouring undeformed region ( Fig. 3b,c ). The corresponding selected area electron diffraction patterns taken from the two regions are nearly identical (the insets of Fig. 3b and c ), indicating that no detectable crystal-to-crystal phase transition takes place during deformation. Interestingly, we found that in the deformed region the B 4 C nanograins, encapsulated by thin amorphous layers, appear to undergo GB sliding during deformation ( Fig. 3d ). The diffusive interface contrast is apparently different from the sharp interfaces in the undeformed region ( Fig. 1 ). No cracks can be found within the residual indentation region, indicating primarily intrinsic toughening of the n-B 4 C. This feature is quite different from the microcrystalline B 4 C in which failure proceeds by cleavage accompanying the formation of a-B 4 C (refs 1 , 26 ). Therefore, the enhanced fracture toughness of the n-B 4 C appears to be associated with the GB sliding along the thin amorphous carbon layers as well as the nanopores by which local plastic deformation by GB sliding can be accommodated to prevent crack initiation [27] , [28] . Figure 3: Evidence of GB sliding within the deformed area. ( a ) TEM micrograph of n-B 4 C sliced from an indented impression made by 1,000-mN applied force. The sliced residual indent was lifted up using FIB and attached to Cu grid. The dash line (red) indicates the profile of the residual indent. Scale bar, 2 μm. ( b ) Bright-field TEM image of undeformed region shows the homogenous distribution of nanoporosity. The inserted is a SAED pattern taken from this region. Scale bar, 500 nm. ( c ) Bright-field TEM image of the deformed area (underneath the indenter) showing the elimination of nanoporosity. The inserted SAED pattern is taken from the deformed region with densely distributed rings owing to increased nanograin density. Scale bar, 500 nm. ( d ) Zoom-in TEM image beneath indenter showing the well-distributed amorphous phases along GBs caused by GB sliding. Scale bar, 50 nm. Full size image The bright-field scanning transmission electron microscopy (STEM) images taken from these deformed regions reveal amorphous nature of the interface phases between B 4 C grains ( Fig. 4 ). Separate electron energy loss spectroscopy (EELS) measurement performed on these interfaces and crystalline B 4 C reveals two types of amorphous interface phases in the deformed sample. In general, the thicker amorphous interface phase contains significant carbon compared with the crystalline B 4 C ( Fig. 4a and b and Supplementary Fig. S4a–c ), whereas the thinner amorphous interface phase has the boron to carbon ratio close to that of the crystalline B 4 C ( Fig. 4c and d and Supplementary Fig. S4d–f ). The former interface phase seems to be associated with the original amorphous carbon at GBs. The amorphous B 4 C could be formed by deformation-induced phase transition at clean B 4 C GBs during GB sliding and nanopore elimination. These observations suggest that the disordered boundary phases have an important role in enhancing the plasticity of the brittle ceramic material by acting as a lubricant to promote GB sliding. 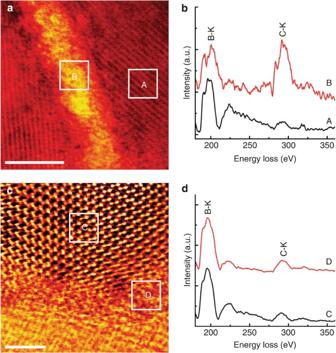Figure 4: Determination of amorphous carbon and a-B4C at interface region using STEM. (a) High-resolution STEM image from indented region at 1,000-mN applied force, showing a wide amorphous interface layer between two B4C grains; Scale bar, 5 nm; and (b) EELS spectra taken from the grain and GB regions (marked as A and B), confirming the amorphous interfacial phase is amorphous carbon (a-C) (red curve) and crystalline B4C (black curve). (c) High-resolution STEM image showing a narrow amorphous interface layer with a width of ~1.4 nm; Scale bar, 2 nm; and (d) EELS spectra taken from both grain and GB areas (marked as C and D), demonstrating the narrow amorphous interfacial phase is amorphous B4C (red curve) with boron and carbon ratio close to that of crystalline B4C (black curve). Figure 4: Determination of amorphous carbon and a-B 4 C at interface region using STEM. ( a ) High-resolution STEM image from indented region at 1,000-mN applied force, showing a wide amorphous interface layer between two B 4 C grains; Scale bar, 5 nm; and ( b ) EELS spectra taken from the grain and GB regions (marked as A and B), confirming the amorphous interfacial phase is amorphous carbon (a-C) (red curve) and crystalline B 4 C (black curve). ( c ) High-resolution STEM image showing a narrow amorphous interface layer with a width of ~1.4 nm; Scale bar, 2 nm; and ( d ) EELS spectra taken from both grain and GB areas (marked as C and D), demonstrating the narrow amorphous interfacial phase is amorphous B 4 C (red curve) with boron and carbon ratio close to that of crystalline B 4 C (black curve). Full size image Micro-compression testing The deformation behaviour of n-B 4 C was further investigated by uniaxial micro-compression testing. The diameters of the pillar specimens are in a range from 1.5 to 7 μm and the aspect ratio is ~2.5:1. 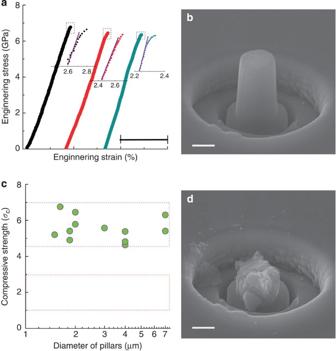Figure 5: Uniaxial micro-compression testing of n-B4C micropillars. (a) Representative engineering stress-strain curves of n-B4C pillars subjected to uniaxial micro-compression at a constant loading rate of 0.33 mN s−1. Typical stress-strain shown for the micropillar diameter of 1.6 μm (black curve), 2 μm (red curve) and 7 μm (dark cyan curve). The inserts show the detectable plastic yielding (~0.08–0.05%) of the pillars with different sizes. Scale bar of strain, 3%. (b) SEM micrograph of a representative n-B4C pillar fabricated by FIB milling, Scale bar, 1 μm. (c) The plot of measured strength values versus the diameter of n-B4C micropillars. All the n-B4C pillars show the failure strength above 4.5 GPa, much higher than that of dense microcrystalline B4C in the strength range marked by the red dotted lines (refs5,29,30). (d) SEM micrograph of a compressed pillar, showing fragmentation via intergranular fracture. Scale bar, 1 μm. Figure 5a shows the representative engineering stress-strain curves of micro-pillars with diameters of 1.6, 2 and 7 μm, respectively. These micropillars were fabricated using FIB milling, and the template SEM image shown is for a 1.6-μm-diameter pillar in Fig. 5b .The fracture strength as the function of sample diameters is plotted in Fig. 5c . It can be seen that for all the micropillars, the strength is above 4.5 GPa and the maximum strength is as high as ~7 GPa, more than two to four times higher than the macroscopic strength and micro-compression strength ( Supplementary Fig. S5 ) of dense bulk microcrystalline B 4 C (1–3 GPa) [5] , [29] , [30] . However, the pillar strength does not have obvious correlation with the sample diameters, indicating the ultrahigh strength, coherent with the hardness, is the intrinsic mechanical property of the n-B 4 C, rather than the sample size effect, which is different from the microcrystalline B 4 C ( Supplementary Fig. S5 ). The variation in strength may arise from the inhomogeneous distribution of the nanopores and weak interface phases. More interestingly, when the high strength of above ~6.5 GPa is achieved, the micropillars, regardless of diameters, exhibit miniature yet obvious plastic strain of ~0.05–0.08% ( Fig. 5a ), which has never been observed in the brittle B 4 C ceramics before. In order to verify this observation, we have carried out micro-compression tests of single-crystal B 4 C with an orientation of (223) and microcrystalline B 4 C prepared by hot pressing [20] . We cannot see any detectable plasticity before failure during uniaxial compression of these micropillars ( Supplementary Fig. S5 ). The failure of the n-B 4 C micropillars is found to proceed in the mode of intergranular fracture, and on the fracture surface no river patterns, characteristic of brittle cleavage in microcrystalline B 4 C [5] , can be observed ( Fig. 5d and Supplementary Fig. S6 ). Raman spectra ( Supplementary Fig. S7 ) from a fractured n-B 4 C micropillar indicate that no obvious crystalline-to-a-B 4 C phase transition occurs during the uniaxial deformation. This is probably owing to relatively low plastic strains imposed on the fractured pillar during uniaxial compression, compared with that in nanoindentation tests. The fractured micropillar surface displays only Raman bands of B 4 C and amorphous carbon, and their corresponding peaks as shown in dotted lines in Supplementary Fig. S7 . The increased intensity of carbon D and G bands at 1360 cm −1 and 1590 cm −1 may be associated with the fact that the fracture surface may expose more interfacial amorphous carbon as the GBs with amorphous carbon are relatively weak and hence can be an easy path for cracking. Figure 5: Uniaxial micro-compression testing of n-B 4 C micropillars. ( a ) Representative engineering stress-strain curves of n-B 4 C pillars subjected to uniaxial micro-compression at a constant loading rate of 0.33 mN s −1 . Typical stress-strain shown for the micropillar diameter of 1.6 μm (black curve), 2 μm (red curve) and 7 μm (dark cyan curve). The inserts show the detectable plastic yielding (~0.08–0.05%) of the pillars with different sizes. Scale bar of strain, 3%. ( b ) SEM micrograph of a representative n-B 4 C pillar fabricated by FIB milling, Scale bar, 1 μm. ( c ) The plot of measured strength values versus the diameter of n-B 4 C micropillars. All the n-B 4 C pillars show the failure strength above 4.5 GPa, much higher than that of dense microcrystalline B 4 C in the strength range marked by the red dotted lines (refs 5 , 29 , 30 ). ( d ) SEM micrograph of a compressed pillar, showing fragmentation via intergranular fracture. Scale bar, 1 μm. Full size image From the micro-indentation and uniaxial compression tests, GB sliding appears to be the underlying mechanism of plastic deformation as well as the enhanced fracture toughness of n-B 4 C. In comparison with the intragranular deformation by twins and dislocations that usually take place in high-strength ceramics under shock loading and high contact pressures or at high temperatures [1] , [31] , [32] , GB sliding in the n-B 4 C is easy to activate because the soft amorphous carbon at GBs can act as a lubricant to advocate the GB deformation. Moreover, the nanopores provide a free space to accommodate the GB plastic strains by the elimination of nanoporosity. Traditionally, porosity and weak interface phases are considered to be detrimental, especially in brittle ceramics, as both of them can initiate catastrophic failure at low stress levels [33] , [34] . However, our study is the first to demonstrate that the interplay between nanopores and weak interface phases in nanocrystalline ceramics can enhance the fracture toughness, engineering strength and even ductility of brittle B 4 C. As the nanopores are much smaller than the critical crack size (~3–5 μm) of brittle B 4 C, even they have a sharp corner, they would not serve as the crack sources and instead increase, rather than decrease, fracture strength when the initiated microcracks are blunted by the nanopore-mediated GB sliding, which is lubricated by the interface amorphous carbon. It is evident in the engineering stress-strain curves that n-B 4 C can sustain ultra-large elastic strain of ~2–3% as well as detectable plastic strain at a stress higher than 6.5 GPa under uniaxial compression. These extraordinary mechanical properties have not been achieved in microcrystalline B 4 C before. This study has shown that strength, plasticity and toughness can be enhanced without obvious compromising in hardness and elastic modulus for one of the most brittle ceramics. The improved plasticity and strength in n-B 4 C indicate an essential role of the interplay between weak GB phases and nanopores via GB sliding. The unique combination of mechanical properties presented here may be particularly promising for potential applications in superhard nanostructured coatings, abrasive cutting tools, high-performance carbide electrodes and armours. These findings also underline the importance of nanostructure in the remarkable and unexpected properties of traditional materials and may pave a new way to design brittle ceramics with improved toughness, plasticity and engineering strength. Sample preparation and XRD analysis Commercially available nanocrystalline boron carbide powders (Tekna Plasma Systems Inc., Canada) with particle size ranging from 40–80 nm were used as the starting material. These powders were die pressed at a pressure of 40 MPa into disc shape with dimensions of φ20 mm×10 mm. After cold isostatic pressing under 200 MPa, the powder compacts were encapsulated with a Pyrex-type glass tube (Iwaki Glass Co., Chiba, Japan) in vacuum at a temperature of ~760 °C. The compacts were coated with BN powders (UH-1 grade, Syowa Denko Co., Tokyo, Japan) before cold isostatic pressing to prevent them from reacting with the glass tube. The capsule was heated at a rate of 13 °C min −1 and kept at a temperature of 800 °C in an argon atmosphere for 20 min. Later, the pressure was increased up to 980 MPa at a rate of 13 MPa min −1 . At a pressure of 980 MPa, the temperature was increased to 1,600 °C and kept for 1 h. The final density of the sintered compacts was determined by the Archimedes' method with deionized water as the immersion medium. Phase identification was performed by XRD (RINT 2200, Rigaku X-ray diffractometer) with Cu Kα radiation. Mechanical testing A dynamic ultra-micro-hardness tester (Shimadzu W201S) equipped with a Berkovich indenter was used to carry out the hardness and fracture toughness measurements at maximum loads ranging from 200 to 1000 mN with a constant loading rate of 7.06 mN s −1 . The micropillars with nominal diameters ranging from 1.5 to 7 μm and an aspect ratio of ~2.5:1 (height:diameter) were prepared by a FIB system (JEOL JIB-4600F). A 40-μm-in-diameter pool where a micropillar resides at the centre was designed to provide a sufficient space for the indenter during a test. These micropillars were loaded in uniaxial compression at a constant loading rate of 0.33 mN s −1 using the dynamic ultra-micro-hardness tester with a 10-μm flat-end Berkovoich indenter. Microstructural characterization Microstructural characterization of the n-B 4 C samples was performed using a micro-Raman spectrometer (Renishaw, UK) with an Ar + laser (excitation wavelength 514.5 nm), SEM (JEOL JIB-4600F) and TEM (JEOL JEM-2100F) equipped with double spherical aberration (Cs) correctors for both the probe-forming and image-forming lenses. The cross-sectional TEM specimens of pristine surface and deformed n-B 4 C were prepared by the lift-out technique using a FIB system for detailed microstructure characterization. Atomic structure of the interfaces in n-B 4 C was investigated using bright-field and high-angle annular dark-field STEM. Elemental mappings of the interfacial phases were obtained by STEM-EELS using a Gatan imaging filter system (Gatan GIF-Tridiem). How to cite this article: Madhav Reddy K. et al . Enhanced mechanical properties of nanocrystalline boron carbide by nanoporosity and interface phases. Nat. Commun. 3:1052 doi: 10.1038/ncomms2047 (2012).